Enhanced spin-triplet superconductivity near dislocations in Sr2RuO4 Superconductors with a chiral p -wave pairing are of great interest because they could support Majorana modes that could enable the development of topological quantum computing technologies that are robust against decoherence. Sr 2 RuO 4 is widely believed to be a chiral p -wave superconductor. Yet, the mechanism by which superconductivity emerges in this, and indeed most other unconventional superconductors, remains unclear. Here we show that the local superconducting transition temperature in the vicinity of lattice dislocations in Sr 2 RuO 4 can be up to twice that of its bulk. This is all the more surprising for the fact that disorder is known to easily quench superconductivity in this material. With the help of a phenomenological theory that takes into account the crystalline symmetry near a dislocation and the pairing symmetry of Sr 2 RuO 4 , we predict that a similar enhancement should emerge as a consequence of symmetry reduction in any superconductor with a two-component order parameter. Sr 2 RuO 4 has attracted much attention recently because it may feature a pairing state hosting Majorana bound states useful for topological quantum computing [1] , [2] , [3] . A large body of experimental data, including that obtained in phase-sensitive measurements [4] , has shown that the layered perovskite Sr 2 RuO 4 is a spin-triplet, odd-parity superconductor [5] , [6] . Assuming that superconductivity in this material is two-dimensional in nature, the fourfold tetragonal crystalline symmetry dictates that the pairing symmetry must be one of the five representations [7] . Among those, only the two-component, p x ±i p y state is consistent with the muon spin rotation [8] and Kerr rotation [9] measurements that suggest the presence of a spontaneous magnetic field in the superconducting state of Sr 2 RuO 4 , making it an electronic analogue [7] of the superfluid 3 He A-phase, and a chiral p -wave superconductor for which a Majorana zero-energy mode bound to the normal core of a half-flux quantum vortex has been predicted [1] , [2] . An important question of interest is what is the microscopic mechanism responsible for such a highly exotic superconducting state. In this regard, models based on ferromagnetic [10] or antiferromagnetic fluctuations [11] , spin-orbit coupling [12] , interaction theory [13] , [14] , Hund’s rule coupling [15] and interplay of charge and spin fluctuations in the one-dimensional bands [16] have been proposed. The debate on these mechanisms is currently ongoing [6] . The eutectic phase of Sr 2 RuO 4 -Ru featuring crystalline islands of Ru embedded in the bulk crystalline Sr 2 RuO 4 , found previously to feature a superconducting transition temperature ( T c ) nearly double than that of the bulk Sr 2 RuO 4 (ref. 17 ), may provide insight into the mechanism issue. The T c enhancement was attributed to the capillary effect at the Ru/Sr 2 RuO 4 interface [18] . It was more recently suggested that the enhanced superconductivity occurs on the Sr 2 RuO 4 side away from [19] rather than at the Ru/Sr 2 RuO 4 interface as assumed previously [18] . Meanwhile, dislocations were found to be abundant, which led to the intriguing question as to whether these dislocations are the origin of the enhancement of T c [19] . The bulk eutectic phase of Sr 2 RuO 4 -Ru possesses both Ru/Sr 2 RuO 4 interfaces and dislocations ( Fig. 1a ), making it difficult to separate the effect of dislocations from that of the interfaces. Single-crystal flakes of Sr 2 RuO 4 prepared by mechanical exfoliation, in which islands of Ru and dislocations can be identified by scanning electron microscopy (SEM) and/or transmission electron microscopy (TEM; Fig. 1b ), provide an opportunity to study separately the respective effect of the Sr 2 RuO 4 /Ru interface and dislocations (see below). Interestingly, an edge dislocation in a Sr 2 RuO 4 lattice ( Fig. 1c ) is expected to possess complicated modifications to the local crystalline structure and electronic states, which may lead to a new way of hosting a Majorana zero mode [20] . Nevertheless, it has a dominating overall feature that the fourfold rotational symmetry is lowered to one that is basically twofold. 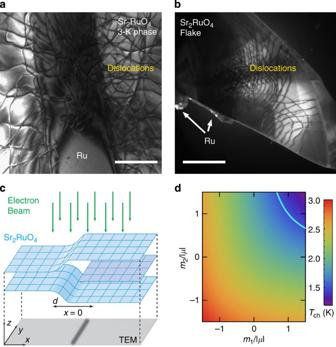Figure 1: Dislocations and prediction of an enhancedTc. (a) Transmission electron microscopy (TEM) image of a Sr2RuO4-Ru eutectic crystal showing a Ru island in the middle and large numbers of dislocations. (b) TEM image of a Sr2RuO4single-crystal flake, showing dislocations and nanodomains of Ru on the edge. The dislocation lines are the superposition of many layers. Scale bars, 500 nm. (c) Schematic of an edge dislocation caused by an extra layer (purple) in a Sr2RuO4lattice, indicating that the local fourfold rotational symmetry is broken. The edge dislocation scatters the electron beam in a TEM study, manifesting itself as a dark line in the TEM image. (d)Tchplotted as a function ofm1/|μ| andm2/|μ| for |μ|/αTc0=0.4. The value ofTchis represented by a colour scale. The highlighted curve represents the contour ofTch=1.5 K. Figure 1: Dislocations and prediction of an enhanced T c . ( a ) Transmission electron microscopy (TEM) image of a Sr 2 RuO 4 -Ru eutectic crystal showing a Ru island in the middle and large numbers of dislocations. ( b ) TEM image of a Sr 2 RuO 4 single-crystal flake, showing dislocations and nanodomains of Ru on the edge. The dislocation lines are the superposition of many layers. Scale bars, 500 nm. ( c ) Schematic of an edge dislocation caused by an extra layer (purple) in a Sr 2 RuO 4 lattice, indicating that the local fourfold rotational symmetry is broken. The edge dislocation scatters the electron beam in a TEM study, manifesting itself as a dark line in the TEM image. ( d ) T ch plotted as a function of m 1 /|μ| and m 2 /|μ| for |μ|/α T c0 =0.4. The value of T ch is represented by a colour scale. The highlighted curve represents the contour of T ch =1.5 K. Full size image Here we report our observation of the enhancement in local T c near lattice dislocations in Sr 2 RuO 4 up to about twice of the bulk. We develop a phenomenological theory to describe the observation and predict that the enhanced T c is ubiquitous for symmetry reduction in superconductors with a two-component order parameter. Phenomenology A phenomenological theory can be formulated to capture the effect of the symmetry reduction. The general free-energy density of the bulk Sr 2 RuO 4 with a fourfold tetragonal symmetry in zero magnetic field can be written as [18] , where η x and η y denote the two-component order parameter, a ( T )=α( T − T c0 ), with α a constant and T c0 =1.5 K the bulk T c of Sr 2 RuO 4 , b i ( i =1–3) and K j ( j =1–5) parameters characterizing the bulk superconductor. The effect of the symmetry lowering near a dislocation can be illustrated by first considering a bulk Sr 2 RuO 4 crystal. When an in-plane uniaxial strain is applied to the crystal, the lattice distortion leads naturally to a structural distortion and change in the electronic band structure, which may in turn cause the T c to change. Without getting into the analysis of the complicated microscopic effect, we will write down a phenomenological theory featuring a set of phenomenological parameters, m 1 and m 2 used to quantify the effect of structural distortions and μ to measure the hybridization of the two-order parameter components, describing the symmetry-breaking strength. To obtain only the highest superconducting transition temperature ( T ch ), it is sufficient to consider the free-energy density up to the quadratic terms. We assume a spatially uniform-order parameter, for which the gradient terms vanish. Therefore, following the idea of degenerate perturbation theory, the free-energy density describing the reduced symmetry ( f RS ) can be written as [21] , [22] The modified transition temperature T ch , determined by the eigenvalues of the quadratic terms, is given by where m ± =( m 1 ± m 2 )/2. Equation (3) indicates that the asymmetry-related terms m − and μ always enhance T ch in one superconducting channel, whereas reduce it in the other. In general, the level of crystalline distortion m + may either enhance or suppress the transition temperature. For certain parameters, the symmetry-lowering effect dominates and T ch > T c0 can be obtained ( Fig. 1d ). The above consideration may be extended to the analysis of a bulk crystal of Sr 2 RuO 4 possessing a single dislocation ( Fig. 1c ). If the dislocation line features a width d in the x direction, we may obtain the local T c from T ch ( m 1 , m 2 and μ) in the above treatment of a bulk crystal subjecting to a uniaxial stress. The effect of the bulk on the embedded dislocation region in this approach is described by a δ-function in the free-energy density as done previously to account for the capillary effect at the interface between Ru and Sr 2 RuO 4 (ref. 18 ). Solving the linearized Ginzburg–Landau equations derived from equation (1) and matching the boundary conditions at x =0 (see Methods), we found that T c is given by the solution of which requires that T ch > T c > T c0 for self consistency. The spatial dependence of the order parameter was found to be symmetric with respect to the dislocation line at x =0, with the order parameter reaching a maximum value at the dislocation below T c . As the highest transition temperature found in any Sr 2 RuO 4 including eutectic systems is 3.2 K (ref. 6 ), we assume that T ch =3.2 K. As a result, the experimentally observed typical onset T c of 2.5 K corresponds to d =3.5( K 2 / α T c0 ) 1/2 . This d -value is comparable to the superconducting coherence length given by ξ 1,2 (0)=( K 1,2 / α T c0 ) 1/2 for the anisotropic stripe, suggesting that the use of a δ-function is self-consistent, given that the basic length for order parameter variation in the Ginzburg–Landau theory is ξ 1,2 (0). It is interesting to note that similar phenomenology can be obtained if two pairing states represented by a single-component order parameter have identical or very close intrinsic T c . We note that the above theory is not applicable for a point defect for which the perturbation to local crystalline structure is essentially isotropic (rotationally invariant). The main predictions of our phenomenological theory are threefold. First, an enhanced T c can be obtained if the symmetry reduction effect dominates over other effects from the presence of a dislocation; second, the resulting local T c depends strongly on the parameters characterizing the symmetry reduction, suggesting that the local T c may vary from dislocation to dislocation; third, the magnitudes of the two components of the superconducting order parameter near a dislocation may depend on the temperature differently, leading to a change in the pairing symmetry as the temperature is lowered (see below). Electrical transport Single-crystal flakes of Sr 2 RuO 4 were selected under optical microscope and examined by SEM before device fabrication. Some flakes were also examined by TEM. Dislocations and Ru nanodomains can be identified. Ru nanodomains (if observed) appear to always locate at the edge of the crystal ( Fig. 1b ), perhaps because cleaving tends to occur at the Ru/Sr 2 RuO 4 boundary because of a reduced mechanical strength. For most flakes, however, SEM imaging did not show any Ru nanodomains. These Ru-free flakes of Sr 2 RuO 4 were used to prepare four-point devices for electrical transport measurements. In particular, the temperature dependence of the resistivity for sample A ( Fig. 2a ) shows an onset T c of 1.45 K ( Fig. 2b ), very close to the optimal T c of Sr 2 RuO 4 . For sample B, SEM imaging revealed no Ru nanodomains ( Fig. 2d ) before the low-temperature transport measurement. However, transport measurements showed an onset T c of 2.8 K ( Fig. 2f ). TEM studies of the same device after the transport measurements confirmed the absence of Ru nanodomains and further revealed the presence of dislocations between the two voltage leads ( Fig. 2e ). Similar results were obtained in sample C ( Fig. 2g,h ) with onset T c =1.9 K ( Fig. 2i ). The magnetic field dependence of the resistivity for field applied along the c axis was also measured. It was found that the upper critical field ( H c2 ) is 50 mT for sample A ( Fig. 2c ), comparable to that of the pure phase (75 mT), whereas sample C showed an H c2 of 0.3T (inset of Fig. 2i ), closer to that of the eutectic phase [5] , [6] . Therefore, our experimental observations provide a direct confirmation that the presence of dislocations leads to the enhancement of T c in Sr 2 RuO 4 as predicted by the theory. 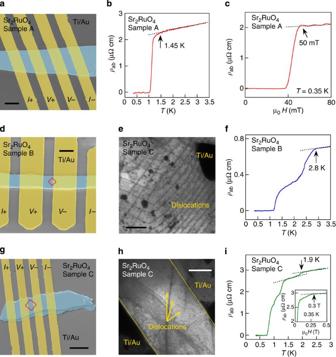Figure 2: Observation of an enhancedTcwith dislocations. (a) False-colour SEM image of sample A. Scale bar, 5 μm. (b) Temperature dependence of the in-plane resistivityρabfor sample A, taken at zero applied magnetic field. (c) Magnetic field dependence ofρabfor sample A. (d) False-colour SEM image of sample B. The red square indicates the area examined by TEM. Scale bar, 5 μm. (e) TEM image of the boxed area indfor sample B, showing dislocation lines but no Ru nanodomains. Scale bar, 200 nm. The regions not shown in this image were also checked by TEM and found to possess no Ru nanodomains. (f) Zero-fieldρab(T) for sample B. (g) False-colour SEM image of sample C. The red square indicates the area examined by TEM. Scale bar, 10 μm. (h) TEM image of the boxed area ingfor sample C. Scale bar, 1 μm. (i) Zero-fieldρab(T) for sample C. Inset:ρab(H) for sample C. In the above line plots, the dashed lines indicate a linear fit of the normal-state resistivity. The deviation from such a fit defines the onsetTcand upper critical field. Figure 2: Observation of an enhanced T c with dislocations. ( a ) False-colour SEM image of sample A. Scale bar, 5 μm. ( b ) Temperature dependence of the in-plane resistivity ρ ab for sample A, taken at zero applied magnetic field. ( c ) Magnetic field dependence of ρ ab for sample A. ( d ) False-colour SEM image of sample B. The red square indicates the area examined by TEM. Scale bar, 5 μm. ( e ) TEM image of the boxed area in d for sample B, showing dislocation lines but no Ru nanodomains. Scale bar, 200 nm. The regions not shown in this image were also checked by TEM and found to possess no Ru nanodomains. ( f ) Zero-field ρ ab ( T ) for sample B. ( g ) False-colour SEM image of sample C. The red square indicates the area examined by TEM. Scale bar, 10 μm. ( h ) TEM image of the boxed area in g for sample C. Scale bar, 1 μm. ( i ) Zero-field ρ ab ( T ) for sample C. Inset: ρ ab ( H ) for sample C. In the above line plots, the dashed lines indicate a linear fit of the normal-state resistivity. The deviation from such a fit defines the onset T c and upper critical field. Full size image The presence of multiple dislocations in our sample, which should be described by different sets of symmetry reduction parameters, should result in multiple phases in the samples with enhanced T c . This is indeed consistent with the multiple features observed in the ρ ab ( T ) curves ( Fig. 2f,i ). Further, the voltage–current ( V–I ) characteristics and the d V /d I – I curves were found to show double features suggesting the existence of two different phases at low temperatures in sample C ( Fig. 3a ), one corresponding to the dislocations and the other the bulk phase. In contrast, in sample A, a single onset T c ( Fig. 2b ) and a single feature ( Fig. 3b ) were found in the ρ ab ( T ), and V–I and d V /d I – I curves, respectively. 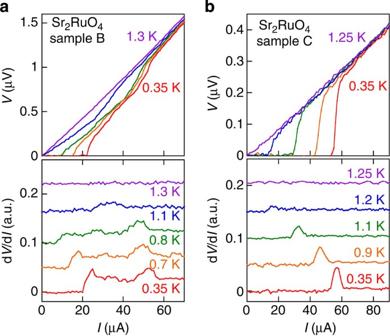Figure 3: Observation of multiple superconducting phases. Zero-fieldV–Icurves and corresponding dV/dI–Icurves at various temperatures for (a) sample C showing multiple transitions and (b) sample A showing a single transition. The dV/dI–Icurves except for those at 0.35 K were shifted for clarity. Figure 3: Observation of multiple superconducting phases. Zero-field V–I curves and corresponding d V /d I – I curves at various temperatures for ( a ) sample C showing multiple transitions and ( b ) sample A showing a single transition. The d V /d I – I curves except for those at 0.35 K were shifted for clarity. Full size image Tunnelling In addition to an enhanced T c and inhomogeneous superconducting phase, the phenomenological theory presented above also predicts that the relative magnitude of the two components of the superconducting order parameter varies strongly as the temperature is lowered. In particular, for a system with an onset T c of 2.5 K, the y component of the order parameter η y was calculated (see Methods) and found to be much larger than the x component η x above T c0 ( Fig. 4a , upper panels) at 1.9 K (below T c ). On the other hand, the two components become comparable below T c0 ( Fig. 4a , lower panels). Therefore, the local density of states (DOSs) near a dislocation should vary accordingly as the temperature is lowered. 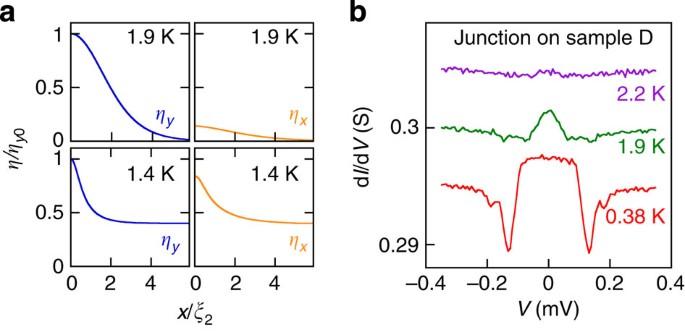Figure 4: Variations of the superconducting order parameter as a function of temperature. (a) Spatial dependence ofηxandηynormalized to the value ofηyatx=0 forT1=1.9 K andT2=1.4 K. Other parameters areTc0=1.5 K,Tch=3.2 K,Tc=2.5 K andξ2(T1,2)=[K2/|α(T1,2−Tc0)|]1/2, superconducting coherence lengths at finite temperatures. (b) Quasiparticle tunneling spectra obtained from the junction on sample D, showing a ZBCP below 2.2 K. The ZBCP at 1.9 K shows a triangular shape, whereas that at 0.38 K shows a rectangular shape. Figure 4: Variations of the superconducting order parameter as a function of temperature. ( a ) Spatial dependence of η x and η y normalized to the value of η y at x =0 for T 1 =1.9 K and T 2 =1.4 K. Other parameters are T c0 =1.5 K, T ch =3.2 K, T c =2.5 K and ξ 2 ( T 1,2 )=[ K 2 /|α( T 1,2 − T c0 )|] 1/2 , superconducting coherence lengths at finite temperatures. ( b ) Quasiparticle tunneling spectra obtained from the junction on sample D, showing a ZBCP below 2.2 K. The ZBCP at 1.9 K shows a triangular shape, whereas that at 0.38 K shows a rectangular shape. Full size image The experimental detection of the temperature dependence of the order parameter near a dislocation is a significant challenge. Ideally, a local probe such as a scanning tunneling microscope with tunneling spectroscopy capability can be used to probe the local superconducting order parameter. However, as a surface probe, a scanning tunneling microscope cannot locate a dislocation embedded inside the crystal. We performed quasiparticle tunneling measurements on a tunnel junction of Sr 2 RuO 4 -TiAl fabricated on a Ru-free flake. Tunneling spectra obtained at an in-plane magnetic field of 40 mT, at which the superconductivity in Al counter electrodes is suppressed, feature zero-bias conductance peaks (ZBCPs). Such ZBCPs were observed in Sr 2 RuO 4 previously [23] , [24] , and linked to the p -wave pairing symmetry. For sample D (onset T c =2.5 K), the ZBCP was visible at 2.2 K, with its shape varying as the temperature is lowered ( Fig. 4b ). The triangularly shaped ZBCP seen at 1.9 K is particularly akin to those found previously in the break junctions of Sr 2 RuO 4 -Ru eutectic crystals above 1.5 K (ref. 23 ) and is consistent with the expectations of our phenomenological theory that predicts that the η y component dominates at 1.9 K with a nearly zero η x component. On the other hand, the ZBCP found at 0.38 K has a rectangular shape, with an onset of superconducting energy gap feature around 0.2 meV, consistent with the weak-coupling value for a T c of 1.5 K and an order parameter with two equal-magnitude components. The crystalline symmetry lowering characterized by the phenomenological parameters manifests itself microscopically as lattice distortions. An edge dislocation demands the existence of both a compressed region and a stretched region extending along the dislocation line ( Fig. 1c ), allowing extended regions of distortions to occur. It is relevant to note a recent uniaxial pressure study on pure Sr 2 RuO 4 that revealed an enhancement of T c up to 3.2 K (onset) and emergence of a continuous distribution of local T c [25] . The enhancement of T c observed in that experiment can be interpreted as a consequence of enhanced interlayer coupling. Indeed, the quantum oscillation measurements carried out under a hydrostatic pressure [26] suggest that the pressure, which lowers T c of Sr 2 RuO 4 , makes the Fermi surface more two-dimensional like, implying that weakening the interlayer coupling reduces T c , consistent with the uniaxial strain result. Meanwhile, the compressed region near a dislocation favours an increased interlayer coupling, suggesting that the observed enhanced T c in Sr 2 RuO 4 near a dislocation may have its origin also in the strengthening of interlayer coupling. Electronically, the symmetry lowering could also lead to changes in the DOSs near the Fermi level as well as the average pairing interaction evaluated over the perturbed Fermi surface, both of which may cause the T c to vary. The change in the DOSs may favour pairing in a specific channel that will result enhancement of T c for that channel, although the pairing interaction that depends on the exact mechanism is yet to be fully understood. The perturbation on the electronic states by a dislocation should be band dependent, which suggests that our result may have implications on the multiple-band superconductivity picture of Sr 2 RuO 4 (refs 16 , 27 ). The implications of our results on other proposed mechanisms for superconductivity in Sr 2 RuO 4 , such as incommensurate fluctuations [11] or Coulomb interactions [13] , [14] , need to be further clarified. Our experimental results on Ru-free flakes of Sr 2 RuO 4 are in agreement with the phenomenological theory, providing the first demonstration of symmetry reduction-induced T c enhancement near a dislocation in a spin-triplet superconductor featuring a two-component order parameter. Our findings have raised an intriguing question on whether it is possible to use symmetry reduction to raise T c in other exotic superconductors described by a two-component superconducting order parameter. This may also be relevant to multiband superconductors for which the magnitudes of the order parameter on different bands are comparable. More experiments are needed to establish this possibility. Phenomenological theory To solve the linearized Ginzburg–Landau equations on the stripe, we adopt constrains for K j used in ref. 18 , K 1 /3= K 2 = K 3 = K 4 >> K 5 . In the geometry we consider, the problem can be simplified into a one-dimensional problem by ignoring the variations along the y and z axis. To examine the onset T c , we consider the linearized Ginzburg–Landau equations derived from equation (1) for x ≠0. For x =0, we assume a fully transparent boundary at which the solutions have to be continuous. Meanwhile, the solutions satisfy the boundary conditions derived from equation (4) The solutions for temperatures above T c0 have the following forms where ξ 1 ( T )=( K 1 /| a| ) 1/2 . where ξ 2 ( T )=( K 2 /| a |) 1/2 . Matching the boundary conditions equations (8) and (9), we obtain the following equations Note that if T ch > T c0 , we always have a solution T c such that T ch > T c > T c0 . Meanwhile, because K 1 /3= K 2 , equation (15) gives a higher instability temperature, indicating that the y component becomes non-zero first. To obtain the spatial dependence of the order parameters, we numerically solve the Ginzburg–Landau equations by taking the phenomenological parameters 2 b 1 =3 b 2 =−3 b 3 =0.4α, T ch =3.2 K, K 1 /α T c0 =3 K 2 /α T c0 =1, the same as those used in ref. 18 . We expand the δ -function in equation (4) into a Gaussian function. The Ginzburg–Landau equations then read where d =3.5( K 2 /α T c0 ) 1/2 =2, giving rise to T c =2.5 K. When x goes to infinite, the solutions decay to zero for T >1.5 K and approach a constant of η x = η y =(− a /4 b 1 ) 1/2 for T <1.5 K. The results are plotted in Fig. 4a . Material Easily cleavable single crystals of Sr 2 RuO 4 were synthesized by the floating-zone method. Because of the high vapour pressure of RuO 2 , excess Ru needs to be added to form a crystal with the correct atomic ratio. In the crystal we used, 10% excess Ru (a reduced amount of Ru overcompensation) was added in the starting rod to suppress the formation of Sr 2 RuO 4 -Ru and Sr 2 RuO 4 -Sr 3 Ru 2 O 7 eutectic phases, both of which were found previously to possess an enhanced T c [17] , [28] . A bulk crystal from this batch was measured and showed a broad transition with a bulk T c around 1.35 K, slightly lower than the optimal T c for Sr 2 RuO 4 . Given that the same starting material with proper Ru overcompensation does yield crystals of Sr 2 RuO 4 with optimal T c , the slightly suppressed bulk T c value is due to structural imperfection rather than an elevated impurity levels in the crystals. Indeed, devices made on flakes of Sr 2 RuO 4 can show an onset T c very close to the optimal. The use of easily cleavable Sr 2 RuO 4 crystals is necessary for this study as superconducting films of Sr 2 RuO 4 are not available, despite an early report of initial synthesis success [29] . To make a TEM sample of Sr 2 RuO 4 flakes, a bulk Sr 2 RuO 4 crystal was sonicated in methanol. Droplets containing tiny flakes of Sr 2 RuO 4 were dripped onto a TEM grid with carbon membrane. After the methanol dried, Sr 2 RuO 4 flakes remained on the carbon membrane. Thin flakes that are electron-transparent were searched and studied by TEM. Flakes with Ru nanodomains on the edge and a large amount of dislocation lines were observed ( Fig. 1b ). Device fabrications We prepared single-crystal flakes with a lateral dimension of roughly 10–50 μm and a thickness of 300–800 nm by mechanical exfoliation. The flakes were transferred onto a Si/SiO 2 substrate with the c axis of the crystal perpendicular to the substrate. A standard four-point probe was prepared by contact photolithography. Electrical leads of 50 nm Ti and 200 nm Au were deposited. After carrying out electric transport measurements at low temperatures, the flakes of sample B and C were further transferred onto a TEM grid using the standard tool of a tungsten tip. TEM study was then carried out on these two samples, revealing dislocations but no Ru nanodomains ( Fig. 2e,h ). To fabricate quasiparticle tunneling devices on flakes, a few more steps than those for four-point transport devices were taken. In particular, 200-nm-thick SiO 2 was first deposited on top of the flakes as a protection layer. Focused ion beam of 30 kV Ga ions was used to carve ramps on the edge of the flakes. Twenty-minute ion mill of 300 V Ar ions was then used to take off the surface layer damaged by high-energy focused ion beam. After photolithography patterning, 5 nm Ti and 200 nm Al were deposited as a counter electrode. The thin Ti layer was used here to improve the adhesion of Al to Sr 2 RuO 4 . Transport measurements Low-temperature direct current measurements were performed in a 3 He refrigerator with a base temperature of 0.35 K. All leads entering the cryostat are shielded and filtered by low-pass resister-capacitor (RC) filters with a 3-dB cutoff frequency of 600 kHz. How to cite this article: Ying, Y. A. et al . Enhanced spin-triplet superconductivity near dislocations in Sr 2 RuO 4 . Nat. Commun. 4:2596 doi: 10.1038/ncomms3596 (2013).